Transgenerational gene silencing causes gain of virulence in a plant pathogen Avirulence ( Avr ) genes of plant pathogens encode effector proteins that trigger immunity in plants carrying appropriate resistance ( R ) genes. The Phytophthora sojae Avr3a gene displays allelic variation in messenger RNA transcript levels. P. sojae strains with detectable Avr3a gene transcripts are avirulent on plants carrying the R -gene Rps 3a, whereas strains lacking Avr3a mRNA escape detection by Rps 3a and are virulent. Here we show non-Mendelian interactions between naturally occurring Avr3a alleles that result in transgenerational gene silencing, and we identify small RNA molecules of 25 nucleotides that are abundant in gene-silenced strains but not in strains with Avr3a mRNA. This example of transgenerational gene silencing is exceptional because it is naturally occurring and results in gain of virulence in a pathogenic organism. Plant pathogens secrete effector proteins to enable disease, but evolution favors host plant immune systems to recognize these factors as cues for activating rapid defence responses that arrest the infection [1] . Effector-triggered immunity in plants is the consequence of signalling events that are determined by resistance ( R ) gene products interacting, directly or indirectly, with pathogen avirulence ( Avr ) effectors. Phytophthora sojae causes stem and root rot of soybean and is a major disease problem that plagues this crop [2] . The P. sojae Avr3a gene encodes a predicted protein of 111 amino acids that includes a signal peptide, a host-targeting motif and a carboxy-terminal effector domain, which are common features of oomycete Avr effectors [3] , [4] , [5] , [6] . Avr3a resides in a 10.8 kilobase (kb) DNA segment that displays copy number variation among P. sojae strains [5] , [6] . Four haplotypes of Avr3a are known and gain of virulence on the R -gene Rps 3a is caused by messenger RNA transcript differences between strains. In crosses between P. sojae strains P6497 ( Avr3a P6497 / Avr3a P6497 ) and P7064 ( Avr3a P7064 / Avr3a P7064 ), avirulence towards Rps 3a plants segregates as a dominant Mendelian trait conditioned by the presence of Avr3a P6497 . Transcripts of Avr3a P6497 but not Avr3a P7064 mRNA are detectable in each of the parental strains and their progeny [5] , [6] . Sequencing of Avr3a alleles and analysis of mRNA transcripts in 17 different P. sojae strains revealed four different haplotypes [6] , but the inheritance behaviour of each of these haplotypes in segregating populations has not been investigated. The present study was intended to test the inheritance Avr3a in P. sojae strains with haplotypes that are different from strains P6497 and P7064. To our surprise, we discovered that genetic outcrosses between P. sojae strains ACR10 and P7076 resulted in transgenerational gene silencing of Avr3a and gain of virulence on soybean plants carrying the Rps 3a gene. Transgenerational gene silencing of Avr3a To determine the inheritance of other Avr3a alleles, we created crosses between P. sojae strains P7076 ( Avr3a P7076 /Avr3a P7076 ) and ACR10 ( Avr3a ACR10 /Avr3a ACR10 ). The strain P7076 is avirulent, whereas strain ACR10 is virulent on Rps 3a plants, and mRNA transcripts are detectable for Avr3a P7076 but not Avr3a ACR10 , as we have previously shown [5] , [6] ( Fig. 1a ). To select hybrid progeny and follow segregation of Avr3a alleles we used co-dominant DNA markers derived from cleaved amplified polymorphic (CAP) fragments, because Avr3a P7076 and Avr3a ACR10 differ in sequence [5] , [6] . 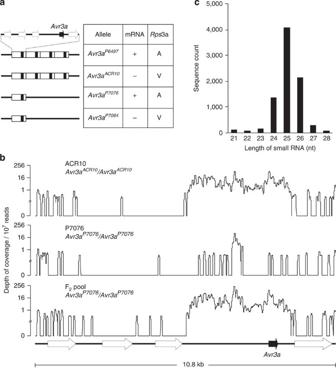Figure 1: Characteristics ofP. sojae Avr3aalleles and deep sequencing of sRNA. (a) A schematic illustration ofAvr3aalleles from four different strains ofP. sojae. The segment of DNA harbouringAvr3aand four other predicted genes is shown. Predicted open reading frames are indicated by bold arrows. Shown for each allele is the copy number of the DNA segment, presence (+) or absence (−) ofAvr3amRNA transcripts and disease outcome onRps3a plants as virulent (V) or avirulent (A). (b) Profiles of sRNA fromP. sojaestrains ACR10 and P7076, and from a pool of F2cultures selected for theirAvr3aP7076/Avr3aP7076genotype. Average depth of coverage across the 10.8-kb genome segment containingAvr3awas normalized to the total number of trimmed reads for each sample. (c) Size of sRNA aligning to the 10.8-kb DNA segment. The total number of counts of RNA sequence reads and the size in nucleotides (nt) is shown forP. sojaestrain ACR10. A total of 28 F 1 hybrid ( Avr3a P7076 /Avr3a ACR10 ) progeny were isolated, scored for virulence on Rps 3a plants and assessed for the presence of Avr3a mRNA transcripts by reverse transcriptase polymerase chain reaction (RT–PCR) ( Table 1 , Fig. 2 , Supplementary Fig. S1 ). All 28 F 1 progeny were virulent on Rps 3a plants and were lacking Avr3a mRNA transcripts. This result was unexpected because heretofore avirulent alleles of Avr3a that accumulate mRNA transcripts were dominant to virulent alleles that lack transcripts, such as in crosses between P. sojae strains P6497 and P7064. To further explore the segregation of Avr3a alleles, virulence and mRNA transcript accumulation in this cross, we generated three different F 2 populations from separate F 1 individuals. In all, 139 F 2 progeny were tested for segregation of Avr3a alleles and mRNA transcripts and scored for virulence on Rps 3a plants. The Avr3a P7076 and Avr3a ACR10 alleles segregated normally in each F 2 population but remarkably all 139 F 2 progeny lacked Avr3a mRNA transcripts and were virulent on Rps 3a plants ( Table 1 ). A sampling of eight F 3 individuals, derived from homozygous Avr3a P7076 /Avr3a P7076 F 2 cultures, indicates that gene silencing is maintained and meiotically stable in these inbred lines ( Supplementary Fig. S2 ). These results demonstrate heritable transgenerational gene silencing of Avr3a in crosses between P. sojae strains ACR10 and P7076. Figure 1: Characteristics of P. sojae Avr3a alleles and deep sequencing of sRNA. ( a ) A schematic illustration of Avr3a alleles from four different strains of P. sojae . The segment of DNA harbouring Avr3a and four other predicted genes is shown. Predicted open reading frames are indicated by bold arrows. Shown for each allele is the copy number of the DNA segment, presence (+) or absence (−) of Avr3a mRNA transcripts and disease outcome on Rps 3a plants as virulent (V) or avirulent (A). ( b ) Profiles of sRNA from P. sojae strains ACR10 and P7076, and from a pool of F 2 cultures selected for their Avr3a P7076 /Avr3a P7076 genotype. Average depth of coverage across the 10.8-kb genome segment containing Avr3a was normalized to the total number of trimmed reads for each sample. ( c ) Size of sRNA aligning to the 10.8-kb DNA segment. The total number of counts of RNA sequence reads and the size in nucleotides (nt) is shown for P. sojae strain ACR10. Full size image Table 1 Segregation of Avr3a alleles and virulence phenotypes in F 1 and F 2 populations (ACR10 × P7076) of Phytophthora sojae. 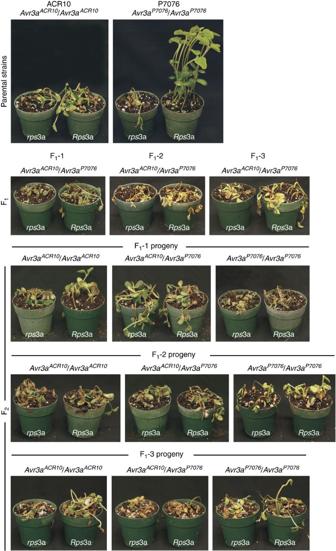Figure 2: Photographs ofP. sojae-infected soybean plants showing disease outcomes. Virulence assays ofP. sojaecultures were performed on greenhouse-grown seedlings of soybean cultivar Williams (rps3a) and the isoline L83-570 (Rps3a) by hypocotyl inoculation withP. sojaemycelia. Shown are disease outcomes 6 days after inoculation of plants with the parental strains, the F1hybrids used to construct each of the three F2populations, or with representative F2individuals illustrating eachAvr3agenotype from the three F2populations tested. Pots are 10 cm in diameter. Full size table Figure 2: Photographs of P. sojae -infected soybean plants showing disease outcomes. Virulence assays of P. sojae cultures were performed on greenhouse-grown seedlings of soybean cultivar Williams ( rps 3a) and the isoline L83-570 ( Rps 3a) by hypocotyl inoculation with P. sojae mycelia. Shown are disease outcomes 6 days after inoculation of plants with the parental strains, the F 1 hybrids used to construct each of the three F 2 populations, or with representative F 2 individuals illustrating each Avr3a genotype from the three F 2 populations tested. Pots are 10 cm in diameter. Full size image Distinctive profile of small RNA (sRNA) in silenced strains To explore the cause of transgenerational silencing of Avr3a , we performed deep sequencing of sRNA from each parental P. sojae strain ACR10 and P7076, and from a sample of F 2 cultures with the genotype Avr3a P7076 /Avr3a P7076 . Results from this analysis show that the profile of sRNA coverage across the Avr3a region differs between ACR10 and P7076 ( Fig. 1b ). The sRNA sequences matching to the Avr3a region are far more abundant in strain ACR10 compared with P7076 ( Table 2 ). The most prevalent of these sRNA molecules are 24–26 nucleotides in length ( Fig. 1c ). In strain ACR10, there is a nearly continuous coverage of sRNA sequences that align to a 3.7 kb span of the Avr3a interval including the 5′ and 3′ intergenic segments but not extending into flanking genes. In contrast, in strain P7076 coverage of matching sRNA is limited to a 0.3-kb segment occurring in the 5′ intergenic region. Sequencing of sRNA from homozygous Avr3a P7076 /Avr3a P7076 F 2 cultures resulted in a profile of coverage that is nearly identical to that from strain ACR10 ( Avr3a ACR10 /Avr3a ACR10 ) rather than that from P7076 ( Avr3a P7076 /Avr3a P7076 ). The sRNA profiles were replicated from independent samples of ACR10, P7076, F 1 and F 2 cultures, and extended to include samples from additional P. sojae strains P6497 and ACR16 ( Table 2 ; Supplementary Fig. S3 ). The results consistently show a pattern of extensive sRNA coverage of Avr3a occurs in gene-silenced strains. Table 2 Deep sequencing of sRNA from Phytophthora sojae. * Full size table Previous studies have shown that transformation of organisms, including species of Phytophthora , with recombinant DNA or RNA molecules can cause internuclear or trangenerational gene silencing that resembles our observations of naturally occurring silencing of Avr3a (refs 7 , 8 ). Moreover, results from comparative genome sequencing of species within the Phytophthora infestans clade suggest a role for epigenetic mechanisms in the rapid evolution of Phytophthora species [9] . Thus, we propose that transgenerational gene silencing of Avr3a in P. sojae is the result of epigenetic changes that modulate the expression state of this gene, and that are transmitted to progeny in a non-Mendelian fashion. Given the emerging functions of sRNAs in controlling epigenetic marks and gene expression states in numerous experimental systems, it is noteworthy that we found an association between sRNAs and gene silencing at the Avr3a locus. In plants, sRNA of 24–26 nucleotides are involved in directing chromatin changes including DNA methylation, whereas shorter ones of 21–22 nucleotides participate in mRNA degradation [10] . Heterochromatic silencing in yeast is initiated by an interaction of sRNA and RNA polymerase II, which guides histone modifications that control chromatin structure and gene expression [11] . Thus, the evidence suggests a role for sRNA in directing the transgenerational gene expression changes of the P. sojae Avr3a gene. Our observations of transgenerational gene silencing of Avr3a provide a remarkable example of pathogen adaptation to host immune surveillance. The interactions between pathogens and their hosts are often interpreted as an evolutionary race, where pathogen virulence and host resistance are at the forefront [12] . Transgenerational gene silencing of an Avr effector locus represents a novel method of host immune evasion that offers the ability to spread quickly in pathogen populations, but yet is potentially reversible as the sequence of the Avr gene itself remains unchanged. We predict that other eukaryotic pathogens of plants, humans and animals will employ similar mechanisms to escape detection by host immune systems. Phytophthora sojae strains and crosses The origin of P. sojae strains and methods of culture, propagation and oospore isolation have been described [5] , [6] , [13] , [14] , [15] . P. sojae is an oomycete and diploid microorganism that reproduces sexually through the development of oogonia (female gametophyte) and antheridia (male gametophyte). P. sojae is homothallic and is not known to have mating types, therefore oospores can develop from self-fertilization or from out-crossing when different strains of the organism are grown together [2] . To perform sexual crosses of P. sojae , parental strains are co-cultivated and oospores are isolated from culture homogenates by a series of purification steps [13] , [14] , [15] . Purified oospores are diluted and plated out on water agar to germinate. Individual germinating oospores are picked under a dissecting microscope and transferred to rich growth medium. Samples of purified DNA from the resulting cultures are tested using co-dominant DNA markers polymorphic between the parents, to determine whether the individuals result from self-fertilization or from out-crossing events between the parental strains. Such markers designed to distinguish Avr3a ACR10 and Avr3a P7076 alleles (described below) were used to identify F 1 progeny in crosses between strain ACR10 and P7076. The F 2 populations were generated by isolating oospores from self-fertilized F 1 individuals. Purification of nucleic acids and scoring of markers and transcripts for Avr3a Mycelia cultures of P. sojae for nucleic acid isolation were grown on vegetable juice (V8) agar media overlaid with cellophane (BioRad). After growth in darkness for 7 days at 25 °C, mycelia-grown cellophane disks were peeled off the media, frozen at −80 °C and ground to a fine powder in liquid N 2 using a mortar and pestle. Genomic DNA was purified using conventional phenol–chloroform extraction procedures followed by precipitation with isopropanol [16] . Purfied DNA pellets were washed with 70% (v/v) ethanol, dried and resuspended in a solution of 10 mM Tris HCl, pH 7.4, 0.1 mM EDTA. CAP markers were used to track segregation of the Avr3a ACR10 and Avr3a P7076 alleles. For CAPs analysis, PCR amplification was performed with 5 ng of genomic DNA as template in a volume of 25 μl under the following conditions: 0.2 mM dNTPs, 1.5 mM MgCl 2 , 0.4 μM of each primer (forward primer 5′-GCTGCTTCCTTCCTGGTTGC-3′ and reverse primer 5′-GCTGCTGCCTTTTGCTTCTC-3′), 1.25 U Taq DNA polymerase and 1 × PCR buffer as recommended by the supplier (Invitrogen, Life Technologies). The amplification was carried out in a 96-well plate (GeneAmp PCR System 9700, Applied Biosystems) under the following conditions: 94 °C for 2 min; 40 cycles of 94 °C for 40 s, 58 °C for 40 s, 72 °C for 2 min; followed by an extension step of 10 min at 72 °C. For restriction analysis of the PCR fragments, 10 μl of the amplified products were incubated overnight at 37 °C in a volume of 20 μl using 3 U of AluI (New England Biolabs). Digestion products were resolved by agarose gel electrophoresis and visualized by ethidium bromide staining according to standard methods [16] . The Avr3a ACR10 sequence includes an Alu I site, whereas the Avr3a P7076 sequence lacks the restriction site and is not digested [5] , [6] . Total RNA was extracted from frozen, pulverized mycelia samples in a solution of phenol-guanidine isothiocyanate (TRIzol, Invitrogen) according to instructions provided by the manufacturer. Approximately 1 μg total RNA was subject to DNaseI (Invitrogen) treatment before RT–PCR, as previously described [5] , [6] . Cycling conditions for detecting transcripts of Avr3a as well as for the P. sojae actin gene (forward primer 5′-CGAAATTGTGCGCGACATCAAG-3′ and reverse primer 5′-GGTACCGCCCGACAGCACGAT-3′), used as a control, were described as above with the exception that 25 cycles were used for transcript analysis. Plant inoculation and virulence assays Virulence assays of P. sojae cultures were performed on greenhouse-grown seedlings of soybean cultivar Williams ( rps ) and the isoline L83-570 ( Rps 3a), according to standard methods [5] , [6] . Soybean seeds (20–30 seeds per pot) were sown in 10 cm pots and grown for 7 days before disease testing. For inoculation, P. sojae cultures were grown for 5–7 days on 0.9% (v/v) V8 agar plates. Inoculum was prepared by excising 1 cm segments of agar cut from the growing edge of mycelia colonies and macerating the cultures through a 3-ml syringe attached to an 18-gauge needle. Soybean plants were inoculated in the mid-section of each hypocotyl by making a small incision for injection of the mycelial slurry. Inoculated plants were covered with plastic bags to maintain humidity for 2 days. Disease symptoms were allowed to develop for an additional 4 days before phenotypes were scored. A minimum of three independent replicates of the disease assay were performed for each P. sojae culture tested. Deep sequencing of P. sojae sRNA To profile sRNA molecules of P. sojae cultures, samples of RNA were purified from mycelia cultures as described above. The size selection of sRNA, attachment of adaptor molecules and library construction was performed using prepared supplies and reagents (Illumina small RNA v1.5), following instructions provided by the manufacturer. Sequencing was performed on a flow cell instrument (Illumina GAII). After trimming to remove adaptor sequences and low-quality sequences, the depth of sRNA coverage of the Avr3a region was determined by alignment, and normalized to the number of reads per library. Average depth of coverage across the 10.8-kb genome segment containing Avr3a was determined using a 50-base pair moving interval and values normalized to the total number of trimmed reads for each sample. The number of trimmed reads obtained for each of the sequenced sRNA libraries is proved in Table 2 . How to cite this article: Qutob, D. et al . Transgenerational gene silencing causes gain of virulence in a plant pathogen. Nat. Commun. 4:1349 doi: 10.1038/ncomms2354 (2013).